Regulated spatial organization and sensitivity of cytosolic protein oxidation inCaenorhabditis elegans Cells adjust their behaviour in response to redox events by regulating protein activity through the reversible formation of disulfide bridges between cysteine thiols. However, the spatial and temporal control of these modifications remains poorly understood in multicellular organisms. Here we measured the protein thiol–disulfide balance in live Caenorhabditis elegans using a genetically encoded redox sensor and found that it is specific to tissues and is patterned spatially within a tissue. Insulin signalling regulates the sensor’s oxidation at both of these levels. Unexpectedly, we found that isogenic individuals exhibit large differences in the sensor’s thiol–disulfide balance. This variation contrasts with the general view that glutathione acts as the main cellular redox buffer. Indeed, our work suggests that glutathione converts small changes in its oxidation level into large changes in its redox potential. We therefore propose that glutathione facilitates the sensitive control of the thiol–disulfide balance of target proteins in response to cellular redox events. The reversible formation of disulfide bonds between cysteine residues is increasingly recognized as an important mechanism for the regulation of protein function. These post-translational modifications can modulate the activity of a wide range of proteins, including transcription factors, kinases, metabolic enzymes and membrane channels [1] , [2] , [3] , [4] , [5] , [6] , [7] . As a result, these modifications affect diverse cellular processes, including metabolism, gene expression and cytoskeletal dynamics [7] , [8] . A better understanding of the mechanisms that control these post-translational modifications in vivo may help to explain why the dysregulation of protein oxidation is a common factor in the development of many chronic diseases, including diabetes, cardiovascular disease, neurodegenerative diseases and cancers [9] , [10] , [11] , [12] . Organisms ranging from bacteria to humans control the formation of protein disulfides in the cytosol through the action of the glutathione and thioredoxin redox systems [13] , [14] . Glutathione (GSH) reduces protein disulfides in a reaction that produces glutathione disulfide (GSSG). Similarly, thioredoxin (trx red ) reduces protein disulfides, in a reaction that produces oxidized thioredoxin (trx ox ). GSSG and trx ox are reduced by NADPH in reactions catalysed by specific enzymes [13] . As a result, the GSH/GSSG and trx red /trx ox couples act as shuttles of electrons between NADPH and protein disulfides [13] . The glutathione and thioredoxin couples have a broad spectrum of distinct but overlapping sets of target proteins [14] . Both of these couples can affect the formation of disulfides within and between proteins. In addition, the glutathione couple also affects the formation of disulfides between proteins and GSH, which are known to modify the activities of a large number of proteins [9] , [10] , [11] , [12] . The tendencies of the glutathione and thioredoxin couples to donate electrons to their target proteins are quantified by their redox potentials. Cellular inputs that affect the relative concentrations of these couple’s oxidized and reduced species will shift their redox potential and tilt the thiol–disulfide balance of their respective protein targets. Thus, knowing the redox potential of these couples can inform us about the thiol–disulfide balance of the network of proteins they control [15] . The human and C. elegans proteomes contain ~210,000 cysteine residues, many of which can form disulfides [15] , [16] . The regulation of protein oxidation under the control of the glutathione couple has remained largely unexplored in multicellular organisms due to the limitations of biochemical approaches that generally do not allow to differentiate between cellular compartments, tissues and even individuals [17] . The recent development of genetically encoded fluorescent redox sensors that respond to the glutathione couple [17] , [18] , [19] , [20] , [21] has enabled studies of the in vivo distribution of this redox potential across subcellular compartments in plants [18] , [19] and across tissues in fruitfly larvae [22] . Here we used this approach to visualize the spatial organization of the glutathione redox potential in the cytosol of live C. elegans and quantify its sensitivity and dynamic response. We found that this redox potential is structured at the tissue and sub-tissue levels, and is regulated by insulin signalling at both of these levels. Notably, our work suggests that the glutathione couple is not positioned to act as a buffer in the cytosol, as its redox potential is highly sensitive even to small changes in glutathione oxidation. This sensitivity may enable cells to respond to small perturbations of their cytosolic redox environment by adjusting the thiol–disulfide balance of the network of proteins controlled by the glutathione couple. Measurement of protein oxidation in vivo To visualize protein disulfide levels with spatial and temporal resolution in live C. elegans , we used the redox probe roGFP1_R12, reduction-oxidation sensitive green fluorescent protein (roGFP) or ‘sensor’ for short [23] . This sensor includes two cysteines whose thiol groups can form a reversible intramolecular disulfide bond. This oxidative modification changes the excitation profile of the sensor’s chromophore by increasing absorption at the 410-nm excitation band and decreasing absorption at the 470-nm band [23] , [24] . The resulting spectral changes allowed us to monitor the balance between reduced (roGFP red ) and oxidized (roGFP ox ) forms of the sensor via ratiometric fluorescence microscopy [24] . We first characterized the response of the sensor in live C. elegans on exposure to exogenous oxidants and reductants that react directly with protein thiols. We treated animals expressing this sensor in the pharyngeal muscles with 50 mM diamide (a thiol-specific oxidant) [25] and then 100 mM dithiothreitol (DTT, a reducing agent), and observed the effect of this treatment time course on the sensor’s fluorescence ( Fig. 1a–d ). Diamide and DTT caused reciprocal changes in fluorescence, indicating that the sensor responds to oxidation and reduction reversibly ( Fig. 1c,d ). This treatment sequence resulted in the maximal oxidation and reduction of the sensor (see Methods). The resulting fluorescence ratio R 410/470 exhibited a large, 7.8-fold dynamic range ( Fig. 1b ). 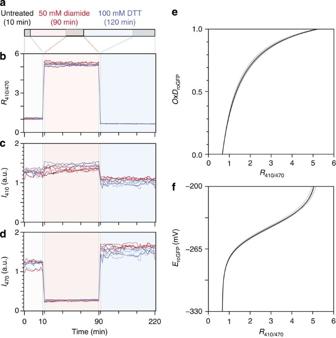Figure 1: Measurement of roGFP1_R12 redox potential in liveC. elegans. (a) Treatment schedule. Each individual was imaged every minute for 10 min before any treatment and during the last 30 min of the diamide and DTT treatments (grey areas in the top bar). (b–d) Fluorescence intensities and ratios for nine individuals in which the sensor was first maximally oxidized and then maximally reduced by diamide and DTT treatments, respectively. (b) RatioR410/470of the fluorescence intensities on excitation with 410 nm (c) and 470 nm (d). (e–f) From theR410/470andI470time courses inbandd, respectively, we determined the three parameters required to relate the fluorescence ratioR410/470to the fraction of roGFP1_R12 molecules with a disulfide bond,OxDroGFP: (i)Rox, the value ofR410/470when the sensor is fully oxidized; (ii)Rred, the value ofR410/470when the sensor is fully reduced; (iii)α=I470(ox)/I470(red), the ratio of fluorescence intensities on excitation with 470 nm when the sensor is fully oxidized and fully reduced. These three parameters enable the conversion ofR410/470toOxDroGFP(ref.17), shown ine:OxDroGFP=(R410/470−Rred)/[α(Rox−R410/470)+(R410/470−Rred)]. The parametersRoxandRreddefine the dynamic range of the sensor (Rox/Rred=7.8). Next, we used the Nernst equation to convertOxDroGFPintoEroGFP, which is the half-cell reduction potential of the sensor redox couple. The parameterαshifts the relationship fromR410/470toEroGFPby a constant value. See Methods for additional considerations. Each of the nine time courses provides one set of three parameters (Rox,Rredandα), yielding a particularOxDroGFPversusR410/470(e) andEroGFPversusR410/470(f) curve. These nine curves are shown in grey. The average value of each parameter (Rox=5.207,Rred=0.667 andα=0.171) yields the curves shown in black that were used throughout the paper to transform our fluorescent readoutR410/470into a biophysically interpretable magnitudeEroGFP. Figure 1: Measurement of roGFP1_R12 redox potential in live C. elegans . ( a ) Treatment schedule. Each individual was imaged every minute for 10 min before any treatment and during the last 30 min of the diamide and DTT treatments (grey areas in the top bar). ( b – d ) Fluorescence intensities and ratios for nine individuals in which the sensor was first maximally oxidized and then maximally reduced by diamide and DTT treatments, respectively. ( b ) Ratio R 410/470 of the fluorescence intensities on excitation with 410 nm ( c ) and 470 nm ( d ). ( e – f ) From the R 410/470 and I 470 time courses in b and d , respectively, we determined the three parameters required to relate the fluorescence ratio R 410/470 to the fraction of roGFP1_R12 molecules with a disulfide bond, OxD roGFP : (i) R ox , the value of R 410/470 when the sensor is fully oxidized; (ii) R red , the value of R 410/470 when the sensor is fully reduced; (iii) α = I 470(ox) / I 470(red) , the ratio of fluorescence intensities on excitation with 470 nm when the sensor is fully oxidized and fully reduced. These three parameters enable the conversion of R 410/470 to OxD roGFP (ref. 17 ), shown in e : OxD roGFP =( R 410/470 − R red )/[ α ( R ox − R 410/470 )+( R 410/470 − R red )]. The parameters R ox and R red define the dynamic range of the sensor ( R ox / R red =7.8). Next, we used the Nernst equation to convert OxD roGFP into E roGFP , which is the half-cell reduction potential of the sensor redox couple. The parameter α shifts the relationship from R 410/470 to E roGFP by a constant value. See Methods for additional considerations. Each of the nine time courses provides one set of three parameters ( R ox , R red and α ), yielding a particular OxD roGFP versus R 410/470 ( e ) and E roGFP versus R 410/470 ( f ) curve. These nine curves are shown in grey. The average value of each parameter ( R ox =5.207, R red =0.667 and α =0.171) yields the curves shown in black that were used throughout the paper to transform our fluorescent readout R 410/470 into a biophysically interpretable magnitude E roGFP . Full size image Although R 410/470 values provide some information about the balance between oxidized and reduced forms of the sensor, they do not represent a biophysically interpretable magnitude. We derived the fraction of sensor molecules with a disulfide bond— OxD roGFP , equal to [roGFP ox ]/([roGFP ox ]+[roGFP red ])—by determining the three conversion parameters relating OxD roGFP and R 410/470 from the fluorescence time courses in diamide- and DTT-treated animals (see Fig. 1e legend and Methods for details). The tendency of roGFP ox to acquire electrons and thereby become reduced into roGFP red is quantified by the half-cell reduction potential of the roGFP red /roGFP ox couple, E roGFP . This redox potential is given by the Nernst equation E roGFP = E roGFP °′ −[ RT /(2 F )] ln ([roGFP red ]/[roGFP ox ]), where R is the gas constant, F the Faraday constant, T the absolute temperature and E roGFP °′ the standard roGFP1_R12 midpoint potential, which is −265 mV (ref. 23 ). Knowing OxD roGFP made it possible to calculate E roGFP by substituting in the Nernst equation the term [roGFP red ]/[roGFP ox ] with the term (1− OxD roGFP )/ OxD roGFP , leading to the relation E roGFP = E roGFP °′ −[ RT /(2 F )] ln [(1− OxD roGFP )/ OxD roGFP ] ( Fig. 1e,f ). Previous studies demonstrate that roGFP-based sensors respond to the glutathione couple via glutaredoxin (see Supplementary Note 1 ). We measured the kinetics of spontaneous recovery from maximal oxidation by transferring animals from diamide treatment back to normal conditions. These in vivo reduction kinetics are fast ( Supplementary Fig. 1 , t 1/2 =4.1 min), and are comparable to those observed in vitro in the presence of glutaredoxin [18] , [19] , [21] . This suggests that the endogenous levels of glutaredoxin are sufficient to ensure the equilibration of the sensor and glutathione couples in pharyngeal muscle. It is noteworthy that the fraction oxidized of roGFP1_R12 and, consequently, the associated redox potential of the sensor couple are in a steady state in untreated animals ( Supplementary Figs 1 and 2 ) and reach a new steady state close to the original on recovery from diamide ( Supplementary Fig. 1 ). The fast kinetics of reduction of the sensor, together with the observed stability in the sensor’s redox potential over time, suggest that the sensor oxidation is in steady state in unperturbed animals because the redox environment controlling its oxidation is stable. To determine whether the sensor responds to changes in the total amount of glutathione in live C. elegans , we measured its redox potential in feeding muscles of animals with reduced gcs-1 activity. The gcs-1 gene encodes the only glutamate–cysteine ligase in the genome, which catalyses the rate-limiting first step in GSH biosynthesis [26] . Animals with reduced gcs-1 activity exhibit lower GSH levels than wild type [26] . The gcs-1(ok436) null allele causes larval lethality; therefore, we examined young (L2) larvae lacking zygotic gcs-1 , derived from gcs-1 heterozygous parents. We found that the sensor’s redox potential was significantly higher in gcs-1(maternal+ zygotic-) animals than in their gcs-1(maternal+zygotic+) siblings ( Supplementary Fig. 3 ). We conclude that roGFP1_R12 responds to changes in GSH synthesis in live C. elegans . The sensor's redox potential varies between tissues To investigate the control of the sensor’s redox potential across tissues of a live animal, we expressed the sensor in the cytosol of cells representing the three primary tissue layers: endoderm (intestine), mesoderm (pharyngeal muscles) and ectoderm (PLM neurons). Unexpectedly, we found that the sensor’s redox potential in each of these tissues varied widely across individuals—up to 13 mV—even though these animals were genetically identical, had the same age and were cultured in the same environment. Despite this individual variation, the sensor’s redox potential differed significantly between these three tissues ( Fig. 2 and Supplementary Fig. 4 ). The intestine had the most oxidizing average redox potential ( E roGFP =−268.1±2.1 mV), followed by the PLM neurons ( E roGFP =−269.9±1.3 mV) and the pharyngeal muscles ( E roGFP =−270.9±1.7 mV). We conclude that the sensor’s redox potential is tissue specific. 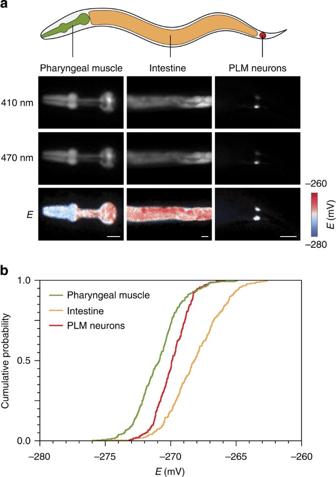Figure 2: Tissue-specific differences in the sensor’s redox potential. (a) Fluorescence images on illumination with 410 and 470 nm for each tissue and pixel-by-pixel redox-potential visualization (scale bar, 25 μm). These animals exhibit potentials close to those of their respective tissue averages. (b) Cumulative distributions of the sensor’s redox potential in the cytosol of pharyngeal muscles (green, 276 animals), PLM touch neurons (red, 239 animals) and intestine (orange, 276 animals), in day 2 adults. Differences in average potential between these tissues were significant (P<0.0001 for all pair-wise comparisons, Tukey HSD test). For statistics seeSupplementary Table 1. Figure 2: Tissue-specific differences in the sensor’s redox potential. ( a ) Fluorescence images on illumination with 410 and 470 nm for each tissue and pixel-by-pixel redox-potential visualization (scale bar, 25 μm). These animals exhibit potentials close to those of their respective tissue averages. ( b ) Cumulative distributions of the sensor’s redox potential in the cytosol of pharyngeal muscles (green, 276 animals), PLM touch neurons (red, 239 animals) and intestine (orange, 276 animals), in day 2 adults. Differences in average potential between these tissues were significant ( P <0.0001 for all pair-wise comparisons, Tukey HSD test). For statistics see Supplementary Table 1 . Full size image The sensor's redox potential is patterned in the pharynx To investigate the spatial control of the sensor’s redox potential within a tissue of a live animal, we chose to focus on the pharynx, the feeding organ of C. elegans ( Fig. 3a ). This large organ has a simple and stereotyped anatomy that facilitates cellular identification. The pharynx is composed of eight adjacent muscles, pm1–pm8, aligned sequentially and connected by gap junctions [27] . We acquired profiles of the sensor’s redox potential along the anterior–posterior (A–P) axis of the pharynx for 394 individuals. We found that these profiles vary considerably across individuals, even though these animals were genetically identical and were cultured in the same environment. At every position along the A–P axis, we observed substantial variation in the sensor’s redox potential between individuals—up to 12 mV ( Fig. 3b ). Within an individual, the sensor’s redox potentials in pm3, pm4, pm5 and pm7 muscles were strongly correlated ( Supplementary Fig. 5 ). Therefore, the sensor’s redox potential varies in a concerted manner throughout the pharynx. 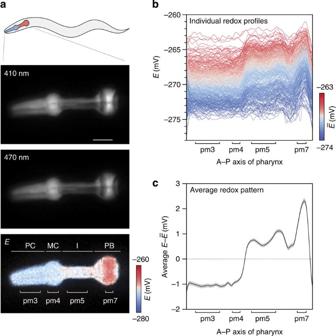Figure 3: The sensor’s redox potential is spatially patterned in the pharynx. (a) Fluorescence images on illumination with 410 and 470 nm of an individual expressing roGFP1_R12 in the pharyngeal muscles (scale bar, 25 μm). The bottom image is a colour-coding of the pixel-by-pixel redox potential, derived from the ratio of the two images above. The annotations in the bottom image indicate the boundaries used to quantify the redox potential of specific muscles: pm3, pm4, pm5 and pm7, which are components of the anatomical regions known as the procorpus (PC), metacorpus (MC), isthmus (I) and posterior bulb (PB), respectively. This animal exhibits a redox potential close to the average for this tissue. (b) This panel shows the redox profiles along the A–P axis of the pharynx of 394 wild-type animals. Each profile is represented as a continuous function in a B-spline basis that best fits the data points (seeSupplementary Methods). The colour of a profile is mapped to its average redox potential . Despite considerable variation in average potential across individuals, most share a distinct redox pattern relative to their tissue mean (c). An alternative representation is given inSupplementary Fig. 6. For statistics seeSupplementary Table 2. (c) Average pharyngeal redox pattern based on the 394 profiles shown inb. A pattern, as distinct from a profile, is defined as the departure of redox potential from the tissue average of an individual (E−). The overall pharyngeal pattern shown here is the average of all individual patterns. The shaded region represents the 95% point-wise confidence interval. Figure 3: The sensor’s redox potential is spatially patterned in the pharynx. ( a ) Fluorescence images on illumination with 410 and 470 nm of an individual expressing roGFP1_R12 in the pharyngeal muscles (scale bar, 25 μm). The bottom image is a colour-coding of the pixel-by-pixel redox potential, derived from the ratio of the two images above. The annotations in the bottom image indicate the boundaries used to quantify the redox potential of specific muscles: pm3, pm4, pm5 and pm7, which are components of the anatomical regions known as the procorpus (PC), metacorpus (MC), isthmus (I) and posterior bulb (PB), respectively. This animal exhibits a redox potential close to the average for this tissue. ( b ) This panel shows the redox profiles along the A–P axis of the pharynx of 394 wild-type animals. Each profile is represented as a continuous function in a B-spline basis that best fits the data points (see Supplementary Methods ). The colour of a profile is mapped to its average redox potential . Despite considerable variation in average potential across individuals, most share a distinct redox pattern relative to their tissue mean ( c ). An alternative representation is given in Supplementary Fig. 6 . For statistics see Supplementary Table 2 . ( c ) Average pharyngeal redox pattern based on the 394 profiles shown in b . A pattern, as distinct from a profile, is defined as the departure of redox potential from the tissue average of an individual ( E− ). The overall pharyngeal pattern shown here is the average of all individual patterns. The shaded region represents the 95% point-wise confidence interval. Full size image Surprisingly, we found that the sensor’s redox potential is not uniform throughout the A–P axis of the pharynx but, instead, is spatially patterned ( Fig. 3c ). We observed three distinct redox regions that align sharply with muscle boundaries ( Supplementary Fig. 6a,b and Supplementary Movie 1 ). These redox regions may encompass multiple muscles, as pm3 and pm4 exhibit no significant difference in the sensor’s redox potential ( Supplementary Fig. 6 ). Along the A–P axis of the pharynx, sensor redox potentials are typically ordered: pm3=pm4<pm5<pm7 ( Fig. 3c and Supplementary Fig. 6 ). Differences between pairs of muscles vary widely between individuals—up to 7.5 mV ( Supplementary Fig. 6c,d and Supplementary Movie 2 ). The redox potential difference between pm3 and pm5 is independent of the difference between pm5 and pm7 ( Supplementary Fig. 7 ), indicating that the redox pattern is generated by two distinct mechanisms. We conclude that the pharyngeal redox profile is patterned by independent mechanisms causing local deviations from the overall glutathione redox potential of the pharynx. Insulin signalling regulates the sensor’s redox potential The well-defined redox pattern we observed in the pharynx and the redox-potential differences we observed across tissues suggest that the sensor’s redox potential may be regulated at the tissue and sub-tissue levels. Insulin signalling has evolutionarily conserved effects on survival under oxidative stress [28] , [29] , making it a good candidate for the modulation of the sensor’s redox potential. We examined mutants of daf-2 , the only insulin receptor gene in C. elegans [30] , and found that they exhibit a more reducing environment in the pharynx. The daf-2(e1370) mutation, which affects the kinase domain of the protein, and the daf-2(m579) mutation, which affects the ligand-binding domain and is homologous to the human type-A insulin resistance mutation [31] , lower the sensor’s redox potential by an average of 2.8 mV ( Fig. 4a and Supplementary Fig. 8 ). We observed similar changes in the intestine of daf-2(e1370) mutants ( Fig. 4b ), but this mutation had no effect on redox potential in the cytosol of PLM neurons ( Fig. 4c ). Thus, under normal conditions, the effect of daf-2 on redox potential is tissue specific. 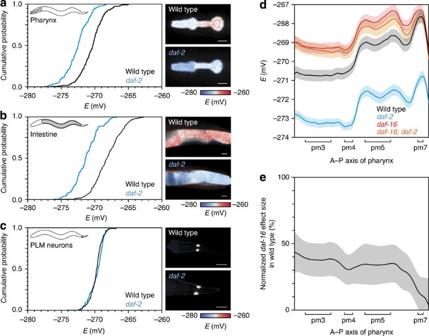Figure 4: Insulin signalling regulates redox potential in different tissues and within a tissue. (a–c) Insulin signalling has tissue-specific effects on cytosolic redox potential. Cumulative distributions of cytosolic redox potentials in wild type anddaf-2(e1370)mutants. The strong inhibition of insulin signalling in thedaf-2(e1370)mutant causes a more reduced environment in the pharynx (a) and intestine (b), but does not affect the redox potential of the PLM touch neurons (c). Pixel-by-pixel redox potential images of representative animals, with potentials close to their respective tissue and genotype averages. Scale bar, 25 μm. Population sizes for wild type anddaf-2(e1370)were, respectively, 227 and 263 (pharynx), 276 and 151 (intestine), and 133 and 205 (PLM neurons). For statistics seeSupplementary Table 3a. (d) Insulin signalling has region-specific effects on the spatial redox profile in the pharynx. We compare the average redox potential along the A–P axis of the pharynx of wild type (black, 273 animals),daf-2(e1370)(blue, 225 animals),daf-16(mu86)(red, 224 animals) and the double-mutantdaf-16(mu86); daf-2(e1370)(orange, 209 animals). The latter two are statistically indistinguishable (P>0.05, functional permutationt-test). Shaded areas represent 95% point-wise confidence intervals. (e) Normalizeddaf-16effect size on the sensor’s redox potential along the A–P axis of the pharynx. We quantify the effect size ofdaf-16on this phenotype using a functional version of categorical regression on genotype. This regression expresses the A–P redox profile in terms of the wild-type profile plus effect terms derived fromdaf-2anddaf-16single and double mutants (Supplementary Fig. 9b,c). In essence, the normalized effect ofdaf-16in wild type is the difference between the black and the red curves divided by the difference between the blue and the orange curves. The latter difference is the maximal effect ofdaf-16controllable bydaf-2. The panel shows that in most of the pharynx of wild-type animalsdaf-16is kept around 40% of its maximal effect, decreasing to 0% in the posterior. The shaded area represents the 95% point-wise confidence interval. Figure 4: Insulin signalling regulates redox potential in different tissues and within a tissue. ( a – c ) Insulin signalling has tissue-specific effects on cytosolic redox potential. Cumulative distributions of cytosolic redox potentials in wild type and daf-2(e1370) mutants. The strong inhibition of insulin signalling in the daf-2(e1370) mutant causes a more reduced environment in the pharynx ( a ) and intestine ( b ), but does not affect the redox potential of the PLM touch neurons ( c ). Pixel-by-pixel redox potential images of representative animals, with potentials close to their respective tissue and genotype averages. Scale bar, 25 μm. Population sizes for wild type and daf-2(e1370) were, respectively, 227 and 263 (pharynx), 276 and 151 (intestine), and 133 and 205 (PLM neurons). For statistics see Supplementary Table 3a . ( d ) Insulin signalling has region-specific effects on the spatial redox profile in the pharynx. We compare the average redox potential along the A–P axis of the pharynx of wild type (black, 273 animals), daf-2(e1370) (blue, 225 animals), daf-16(mu86) (red, 224 animals) and the double-mutant daf-16(mu86); daf-2(e1370) (orange, 209 animals). The latter two are statistically indistinguishable ( P >0.05, functional permutation t -test). Shaded areas represent 95% point-wise confidence intervals. ( e ) Normalized daf-16 effect size on the sensor’s redox potential along the A–P axis of the pharynx. We quantify the effect size of daf-16 on this phenotype using a functional version of categorical regression on genotype. This regression expresses the A–P redox profile in terms of the wild-type profile plus effect terms derived from daf-2 and daf-16 single and double mutants ( Supplementary Fig. 9b,c ). In essence, the normalized effect of daf-16 in wild type is the difference between the black and the red curves divided by the difference between the blue and the orange curves. The latter difference is the maximal effect of daf-16 controllable by daf-2 . The panel shows that in most of the pharynx of wild-type animals daf-16 is kept around 40% of its maximal effect, decreasing to 0% in the posterior. The shaded area represents the 95% point-wise confidence interval. Full size image Next, we determined whether insulin signalling regulates the spatial redox pattern of the pharynx. We acquired A–P profiles of the sensor’s redox potential in mutants of the FOXO transcription factor DAF-16 whose activity is negatively modulated by signalling through DAF-2 (refs 32 , 33 ). We found that daf-16(mu86) null mutants exhibit higher redox potentials in the anterior muscles pm3 and pm5 than wild-type animals ( Fig. 4d and Supplementary Fig. 9a ). However, this mutation does not affect the sensor’s redox potential in the posterior muscle pm7 ( Fig. 4d and Supplementary Fig. 9a ). Thus, in wild-type animals, DAF-16 is partially enabled in the anterior muscles of the pharynx and effectively switched off in the posterior. We also found that daf-2(e1370) lowers the sensor’s redox potential at all positions along the pharyngeal A–P axis ( Fig. 4d and Supplementary Fig. 9a ). This effect is mediated by daf-16 , as the redox profiles of the daf-16 single mutants and daf-16; daf-2 double mutants are indistinguishable ( Fig. 4d and Supplementary Fig. 9a ). We conclude that in contrast to the wild-type case, DAF-16 is enabled in all positions along the A–P axis of the pharynx in daf-2(e1370) mutants. We quantified the relative magnitude of the genetic interaction between daf-2 and daf-16 in the control of the spatial variation of redox potential along the pharyngeal A–P axis using a functional version of categorical regression on genotype [34] ( Fig. 4e ). This analysis indicates that the quantitative regulation of DAF-16 by DAF-2 contributes to the redox pattern of the pharynx. Glutathione does not act as a redox buffer in the cytosol As we noted above, the fast kinetics of reduction and the stability of the sensor’s redox potential indicate that this potential equals the redox potential E GSH of the cytosolic glutathione couple, under unperturbed conditions ( Supplementary Figs 1 and 2 and Supplementary Note 1 ). Glutathione is the most abundant cellular thiol and is widely considered to act as the main redox buffer of the cell [1] , [35] , [36] . Based on this framework, we were surprised to observe a large E GSH variation between individuals ( Figs 2b and 3b ), as this variation is likely to cause significant differences in the thiol–disulfide balance of proteins targeted by the glutathione system (see sensitivity section below). This prompted us to re-examine the notion that the glutathione couple acts as a redox buffer. If the glutathione couple acts as a redox buffer, then its redox potential should have a low sensitivity to changes in the balance between reduced and oxidized glutathione species [37] . We therefore determined whether the redox potentials we measured are located in a region of the Nernst curve where glutathione could be expected to act as a buffer of redox potential. As the oxidation of GSH into GSSG is a bimolecular reaction, E GSH depends not only on the oxidation state of the glutathione couple ( OxD GSH ), that is, the amount of glutathione in its oxidized form (2[GSSG]) relative to total glutathione ( GSH tot =[GSH]+2[GSSG]), but also explicitly on total glutathione GSH tot . To determine OxD GSH , we assumed physiologically plausible values for GSH tot in the range of 1–20 mM, with 10 mM being at the high end of physiological estimates [38] . We placed the E GSH values we measured in the cytosol of cells in the pharynx, intestine and PLM neurons ( Figs 2b and 3b ) in the context of Nernst curves for different values of GSH tot . All of these redox potentials fall in a highly sensitive, non-buffering region of the Nernst curve, where even slight changes in OxD GSH lead to large changes in E GSH ( Fig. 5a ). For example, in a cell that exhibits the average cytosolic E GSH of pm3 muscles (−270 mV), the value of OxD GSH would be 0.0019 assuming a GSH tot of 10 mM. The sensitivity of E GSH to changes in OxD GSH (the slope of the Nernst curve) around this OxD GSH value is 88 times higher than it would be if the glutathione couple were best positioned to buffer redox potential ( Fig. 5b ). This relative sensitivity rises to 696-fold if we assume that GSH tot is 1 mM, at the low end of physiological estimates. We conclude that the glutathione couple does not act as a buffer of redox potential, as previously thought. 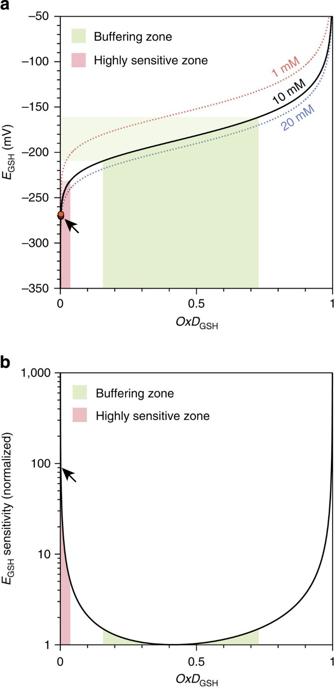Figure 5: The cytosolic glutathione couple is not a buffer of redox potential. (a) The redox potential of glutathione thiol (GSH)/glutathione disulfide (GSSG) couple is given by the Nernst equationEGSH=EGSH°’−[RT/(2F)] ln ([GSH]2/[GSSG]), whereRis the gas constant,Fis the Faraday constant andTis the absolute temperature, here 295.15 °K. The midpoint (standard) potentialE°’for the glutathione couple is −240 mV under biological standard conditions35. This equation can be rewritten in terms of total glutathioneGSHtot(equal to 2 [GSSG]+[GSH]) and the fraction of oxidized glutathioneOxDGSH(equal to 2 [GSSG]/GSHtot), resulting in the expressionEGSH=EGSH°’−[RT/(2F)] ln [2GSHtot(1−OxDGSH)2/OxDGSH]. The panel shows the Nernst curves forGSHtot=1, 10 and 20 mM. A value of 10 mM is at the high end of physiological concentrations observed in other species38. Changes in the oxidation state of the glutathione couple will cause a large change in redox potential when the couple is in a highly sensitive (red) region of the curve and will cause a small change in redox potential when the couple is in a buffered (green) region of the curve. The coloured circles indicate the intersection of the average cytosolic redox potentials we measured in the pharyngeal muscles, intestine and PLM touch neurons (Fig. 2) with the 10-mMGSHtotcurve. (b) Normalized sensitivity of the redox potentialEGSHto changes inOxDGSH(defined as the derivative of the Nernst curves shown ina, normalized to its minimum value).EGSHsensitivity is independent ofGSHtot. Normalized sensitivity values below 1.5 indicate that the glutathione couple operates in a buffering regime (0.157<OxDGSH<0.729, green), while values above 5 indicate a highly sensitive regime (OxDGSH<0.037, red;OxDGSH>0.929, not highlighted). The glutathione couple operates in a highly sensitive regimein vivo(for example, atOxDGSH=0.0019 associated withE=−270 mV, black arrow). This result holds for GSH tot values up to 1 M. Figure 5: The cytosolic glutathione couple is not a buffer of redox potential. ( a ) The redox potential of glutathione thiol (GSH)/glutathione disulfide (GSSG) couple is given by the Nernst equation E GSH = E GSH °’ −[RT/(2F)] ln ([GSH] 2 /[GSSG]), where R is the gas constant, F is the Faraday constant and T is the absolute temperature, here 295.15 °K. The midpoint (standard) potential E °’ for the glutathione couple is −240 mV under biological standard conditions [35] . This equation can be rewritten in terms of total glutathione GSH tot (equal to 2 [GSSG]+[GSH]) and the fraction of oxidized glutathione OxD GSH (equal to 2 [GSSG]/ GSH tot ), resulting in the expression E GSH = E GSH °’ −[RT/(2F)] ln [2 GSH tot ( 1−OxD GSH ) 2 / OxD GSH ]. The panel shows the Nernst curves for GSH tot =1, 10 and 20 mM. A value of 10 mM is at the high end of physiological concentrations observed in other species [38] . Changes in the oxidation state of the glutathione couple will cause a large change in redox potential when the couple is in a highly sensitive (red) region of the curve and will cause a small change in redox potential when the couple is in a buffered (green) region of the curve. The coloured circles indicate the intersection of the average cytosolic redox potentials we measured in the pharyngeal muscles, intestine and PLM touch neurons ( Fig. 2 ) with the 10-mM GSH tot curve. ( b ) Normalized sensitivity of the redox potential E GSH to changes in OxD GSH (defined as the derivative of the Nernst curves shown in a , normalized to its minimum value). E GSH sensitivity is independent of GSH tot . Normalized sensitivity values below 1.5 indicate that the glutathione couple operates in a buffering regime (0.157< OxD GSH <0.729, green), while values above 5 indicate a highly sensitive regime ( OxD GSH <0.037, red; OxD GSH >0.929, not highlighted). The glutathione couple operates in a highly sensitive regime in vivo (for example, at OxD GSH =0.0019 associated with E= −270 mV, black arrow). Full size image As an independent confirmation of this finding, we evaluated recent measurements of glutathione oxidation in C. elegans derived from studies that did not involve genetically encoded sensors. These biochemical measurements on whole-worm extracts directly yield OxD GSH values of 0.028 (ref. 39 ) to 0.035 (ref. 40 ). These extracts average OxD GSH over all cellular compartments, including the highly oxidizing endoplasmic reticulum, where OxD GSH equals 0.4 (ref. 41 ). It is not surprising, therefore, that these reported values are higher by an order of magnitude than the in vivo values we obtained with our targeted cytosolic sensor. Still, even if cytosolic OxD GSH were equal to the values derived from whole-worm extracts, glutathione redox potential would not be buffered ( Fig. 5 ). Glutathione oxidation varies between individuals What are the mechanisms that cause isogenic animals to have different sensor’s redox potentials? The observed differences in redox potential between individuals could be explained by individual differences in the fraction of oxidized glutathione. However, they could also be due to individual differences in total glutathione content. The properties of the Nernst curve allow us to determine which of these two scenarios is dominant, because changes in glutathione oxidation state affect sensitivity (the slope of the Nernst curve, Fig. 5b ), whereas changes in total glutathione do not affect sensitivity at any glutathione oxidation state (they only shift the Nernst curve vertically, Fig. 5a ). To distinguish between these possibilities, we determined whether the magnitude of the animal’s redox response on shift to a more oxidative environment is predicted by the redox potential of the glutathione couple before such shift. If differences in total glutathione were the main source of redox potential variation across individuals, the sensitivities associated with different redox potentials would exhibit little or no variation and, therefore, we would not observe a correlation between redox potential and redox displacements on oxidative shift. On the other hand, if the variation in redox potential across individuals stemmed from differences in the fraction of oxidized glutathione, we would observe a negative correlation between redox potential and the change in redox potential on oxidative shift. In the absence of this Nernst framework, the latter case appears counterintuitive, as it states that animals with higher levels of protein oxidation before oxidant exposure would be less sensitive to oxidant treatment than animals with lower initial oxidation levels. We recorded time series of the sensor’s redox potential in the pharynx of 64 individuals before and after shifting them to media containing 5 mM tert -butyl hydroperoxide ( t -BuOOH). This oxidant does not react with protein thiols directly [42] ; rather, it is thought to act by oxidizing GSH into GSSG, which, in turn, leads to the formation of a disulfide bond within roGFP1_R12. A representative spatiotemporal series shows that different regions along the A–P axis of the pharynx exhibit distinct responses ( Fig. 6a ). We quantified the time-dependent change in the sensor’s redox potential of pm3, pm5 and pm7 muscles relative to their baseline redox potential (defined as the average redox potential before oxidant exposure; Fig. 6b–d and Supplementary Fig. 10 ). Each of these muscles exhibits a distinct response ( Fig. 6e ). Although all muscles experience an increase in the sensor’s redox potential after oxidant exposure, only pm5 and pm7 exhibit an adaptive response consisting of a rise and subsequent decrease in redox potential. In addition to these regularities in the response behaviour of each muscle, we observed a substantial variation across individuals in the magnitude of the response to oxidant treatment ( Fig. 6b–d , and Supplementary Figs 10 and 11 ). Animals with a higher baseline (coloured in red, Fig. 6b–d and Supplementary Fig. 10 ) exhibit smaller redox displacements than animals with a lower baseline (coloured in blue). This relation is confirmed by the negative sign of the observed strong correlations between baselines and early redox displacements of pm3, pm5 and pm7 muscles ( Fig. 6f ). Thus, the response dynamics that we observe indicate that differences in baseline across individuals are due in large part to differences in glutathione oxidation, not glutathione content. 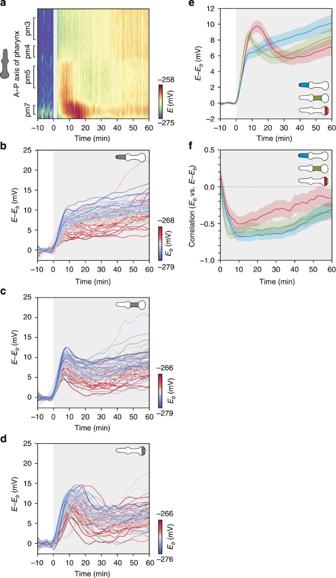Figure 6: Variation in glutathione redox potential between individuals is caused by differences in glutathione oxidation. (a) Spatial and temporal response of the sensor’s redox potential in an individual before and during treatment with 5 mMt-BuOOH. Each column represents the redox profile of the individual along the A–P pharyngeal axis at a given time point. Each row is a time point at a given spatial location. Worms were imaged every 30 s. Oxidant exposure starts att=0 (grey background inb–f). (b–d) The spatiotemporal response to 5 mMt-BuOOH treatment was recorded in 64 individuals. For each individual, we determined the responses of pm3, pm5 and pm7 (b,candd, respectively). Each time series was baseline corrected by subtracting its average potential before oxidant exposure. The resulting time series were converted into a continuous function using a spline basis (for the non-baseline corrected set seeSupplementary Fig. 10; for the quality of the fit seeSupplementary Fig. 11). The colouring encodes the average potential before oxidant exposure (Eb). (e) Average response dynamics. The functionalized trajectories of redox potential in pm3 (blue), pm5 (green) and pm7 (red) were pooled and subjected to functional categorical regression34on the regions of origin (pm3, pm5 and pm7). This procedure yields the average time-dependent response dynamics in each region. Shaded areas represent 68% point-wise confidence intervals. (f) For each muscle, the Pearson correlation between the individual redox baselines before perturbation and the baseline-corrected response after perturbation. The strong initial negative correlation implies that we mostly see different baseline potentials on the same Nernst curve rather than different curves corresponding to distinct values of total glutathione (see text for details). The subsequent correlation decay indicates that an adaptive response to perturbation is becoming prominent. Shaded areas represent 68% point-wise confidence intervals. Figure 6: Variation in glutathione redox potential between individuals is caused by differences in glutathione oxidation. ( a ) Spatial and temporal response of the sensor’s redox potential in an individual before and during treatment with 5 mM t -BuOOH. Each column represents the redox profile of the individual along the A–P pharyngeal axis at a given time point. Each row is a time point at a given spatial location. Worms were imaged every 30 s. Oxidant exposure starts at t= 0 (grey background in b – f ). ( b – d ) The spatiotemporal response to 5 mM t -BuOOH treatment was recorded in 64 individuals. For each individual, we determined the responses of pm3, pm5 and pm7 ( b , c and d , respectively). Each time series was baseline corrected by subtracting its average potential before oxidant exposure. The resulting time series were converted into a continuous function using a spline basis (for the non-baseline corrected set see Supplementary Fig. 10 ; for the quality of the fit see Supplementary Fig. 11 ). The colouring encodes the average potential before oxidant exposure ( E b ). ( e ) Average response dynamics. The functionalized trajectories of redox potential in pm3 (blue), pm5 (green) and pm7 (red) were pooled and subjected to functional categorical regression [34] on the regions of origin (pm3, pm5 and pm7). This procedure yields the average time-dependent response dynamics in each region. Shaded areas represent 68% point-wise confidence intervals. ( f ) For each muscle, the Pearson correlation between the individual redox baselines before perturbation and the baseline-corrected response after perturbation. The strong initial negative correlation implies that we mostly see different baseline potentials on the same Nernst curve rather than different curves corresponding to distinct values of total glutathione (see text for details). The subsequent correlation decay indicates that an adaptive response to perturbation is becoming prominent. Shaded areas represent 68% point-wise confidence intervals. Full size image Sensitivity of protein oxidation to E GSH variation In our study we encountered differences in the sensor’s redox potential across individuals (13 mV), across tissues (2.8 mV), within tissues (7.5 mV), across genetic perturbations (4.2 mV) and under oxidative stress (15 mV). To understand how much these differences may impact protein oxidation, we considered the effect of E GSH variation on the thiol–disulfide balance on protein targets in equilibrium with the glutathione couple. Changes in the glutathione redox potential sway the oxidation states of target proteins in the same direction, but the magnitude depends on both the protein’s tendency to remain reduced (quantified by its midpoint potential) and its initial oxidation state (determined by the redox potential it was experiencing). Midpoint potentials are presently unknown for most proteins. Still, we can treat them as variables and analyse the impact of a redox-potential change on protein oxidation, both in terms of absolute differences and fold changes ( Fig. 7 ). For example, a difference in glutathione redox potential of 10 mV that we typically observe in response to 5 mM t -BuOOH treatment would affect the oxidized fraction of a protein by at most 19% (absolute difference; Fig. 7b ) or by a factor of at most 2.2 (fold change; Fig. 7c ). Such changes can be biologically significant, especially given the wide variety of redox-sensitive proteins. 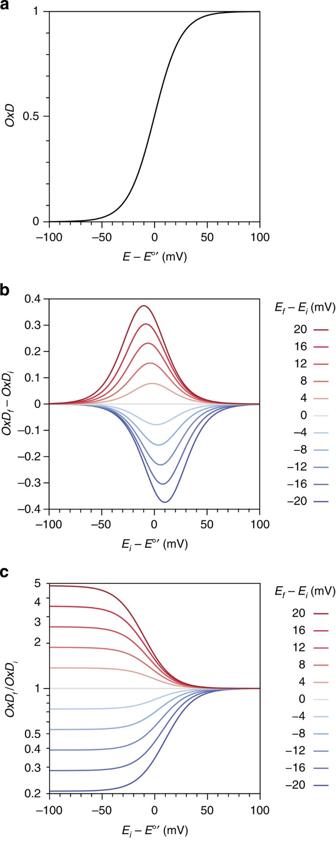Figure 7: Analysis of the sensitivity of protein oxidation to changes in glutathione redox potential. (a) Relationship between redox potential and protein oxidation. The Nernst equation relates the redox potentialEto the fraction oxidizedOxDof a redox couple. This relation depends on the couple’s midpoint potentialE°’(which quantifies the affinity for electrons of the oxidized species). The panel depicts the Nernst curve relative to the midpointE°’, that is,OxDversusE−E°’, withOxD=1/(exp[−(E−E°’)2F/RT]+1) andT=295.15 °K. SeeSupplementary Note 2for additional considerations. (b) Effect of a redox-potential change on absolute protein oxidation levels. The calculation of the change inOxDon a change in potential fromEi−E°’toEf−E°’(that is,ΔE=Ef−Ei), depends on whether the relevant biochemical quantity is the ensuing differenceOxDf−OxDi(this panel) or fold-changeOxDf/OxDi(c). The abscissa shows the initial redox potentialEiof a protein relative to its midpointE°’. The potentialEientails a certain fraction of oxidized proteinOxDi. When the potential changes fromEitoEf, the fraction of protein oxidized changes accordingly fromOxDitoOxDf. This change is reported by the various curves, one for each potential differenceΔE=Ef−Eishown in the legend. (c) Effect of a redox-potential change on relative protein oxidation levels. Similar tob, but the change of interest is now the ratio ofOxDfatEftoOxDiatEi. Note that this is a log-linear plot. The largest fold-change occurs when the initialOxDis as small as possible, as then even the smallest change inOxDresults in a dramatic fold change. This occurs at very negativeEivalues, far to the left of the midpoint. The fold change will be very large (very small) for positive (negative)ΔE. If the protein couple is far to the right of the midpoint,OxDis near maximal and only small changes can occur, resulting in a fold change close to 1. Figure 7: Analysis of the sensitivity of protein oxidation to changes in glutathione redox potential. ( a ) Relationship between redox potential and protein oxidation. The Nernst equation relates the redox potential E to the fraction oxidized OxD of a redox couple. This relation depends on the couple’s midpoint potential E °’ (which quantifies the affinity for electrons of the oxidized species). The panel depicts the Nernst curve relative to the midpoint E °’ , that is, OxD versus E−E °’ , with OxD =1/(exp[ − ( E − E °’ )2 F/RT ]+1) and T =295.15 °K. See Supplementary Note 2 for additional considerations. ( b ) Effect of a redox-potential change on absolute protein oxidation levels. The calculation of the change in OxD on a change in potential from E i −E °’ to E f −E °’ (that is, ΔE = E f − E i ), depends on whether the relevant biochemical quantity is the ensuing difference OxD f −OxD i (this panel) or fold-change OxD f /OxD i ( c ). The abscissa shows the initial redox potential E i of a protein relative to its midpoint E °’ . The potential E i entails a certain fraction of oxidized protein OxD i . When the potential changes from E i to E f , the fraction of protein oxidized changes accordingly from OxD i to OxD f . This change is reported by the various curves, one for each potential difference ΔE = E f −E i shown in the legend. ( c ) Effect of a redox-potential change on relative protein oxidation levels. Similar to b , but the change of interest is now the ratio of OxD f at E f to OxD i at E i . Note that this is a log-linear plot. The largest fold-change occurs when the initial OxD is as small as possible, as then even the smallest change in OxD results in a dramatic fold change. This occurs at very negative E i values, far to the left of the midpoint. The fold change will be very large (very small) for positive (negative) ΔE . If the protein couple is far to the right of the midpoint, OxD is near maximal and only small changes can occur, resulting in a fold change close to 1. Full size image The study of the regulation of cytosolic glutathione redox potential has been challenging, especially in live multicellular organisms. The methods used until recently required the homogenization of samples, resulting in the mixing of subcellular compartments, cells, tissues and often entire populations. In this study, we overcame this difficulty by using a genetically encoded protein sensor. The ability to visualize and quantify the sensor’s redox potential in live individuals, at cellular and high temporal resolution, made it possible to investigate the structure and regulation of the cytosolic glutathione redox potential, as well as the determinants of its variation. As we discuss below, this variation reflects, in part, the high sensitivity of this potential to changes in glutathione oxidation. The regulation of the sensor’s redox potential is suggested by (i) differences in the average redox potentials of the pharynx, intestine and PLM neurons; (ii) the spatial patterning of the sensor’s redox potential along the A–P axis of the pharynx; and (iii) differences in the response dynamics to oxidant treatment of individual pharyngeal muscles. We found that the action of insulin signalling affects the spatial organization of the sensor’s redox potential. The insulin receptor DAF-2 regulates this redox potential in the cytosol in a tissue-specific manner, affecting it in pharyngeal muscles and intestine, but not in PLM neurons. In addition, DAF-2 contributes quantitatively to the spatial patterning of redox potential in the pharynx by regulating the activity of the FOXO transcription factor DAF-16. We also found that a daf-2 mutation that causes type-A insulin resistance in humans is sufficient to lower the cytosolic redox potential of the glutathione couple, which may lead to a significant decrease in the oxidation of target proteins. It would be interesting to investigate whether similar changes in the thiol–disulfide balance are important to the pathogenesis of insulin resistance and diabetes in humans. Glutathione has been widely thought to act as the main redox buffer of the cell [1] , [35] , [36] , a function that provides homeostasis by protecting proteins from the indirect oxidizing action of reactive oxygen species. This view seemed difficult to reconcile with the considerable variation in glutathione redox potential across isogenic individuals, as this variation might cause significant differences in protein oxidation levels. In an effort to substantiate whether the glutathione couple acts as a redox buffer in the cytosol, we found that it does the opposite. The notion of glutathione as a redox buffer may have gained traction over the last half century, because the abundant GSH restores protein thiols that underwent oxidative attack and reduces oxidants such as hydrogen peroxide. Yet, this very action produces an oxidant, GSSG. As most cytosolic glutathione is reduced in vivo , an ever so slight change in GSSG concentration strongly affects the glutathione redox potential ( Fig. 5 ) [43] . Changes in the glutathione redox potential will have repercussions on a much wider array of cysteine thiols than those that were initially threatened by oxidative attack, because cysteine thiols generally react in vivo very slowly with hydrogen peroxide but much faster with GSSG [42] , [44] . Our results call for a change in perspective on the role of the cytosolic glutathione couple. Numerous redox couples, including H 2 O 2 /H 2 O and NADP + /NADPH, interact with the glutathione couple. As a result, the relative levels of GSH and GSSG are determined by a wide range of concurrent processes, including those that generate hydrogen peroxide and those that influence the production or utilization of NADP + and NADPH. As the glutathione couple is not positioned to buffer its redox potential in the cytosol, this potential responds sensitively to changes in glutathione oxidation. We therefore propose that the glutathione couple integrates and amplifies the effects of diverse redox inputs into a single physiological signal: the glutathione redox potential ( Fig. 8 ), to which proteins with embedded cysteines can respond differentially. 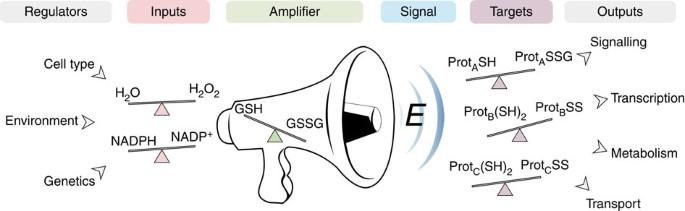Figure 8: Model for redox control of protein function in the cytosol. The cytosolic glutathione couple is positionedin vivoto sensitively amplify redox events affecting its oxidation state, via its redox potentialE. This signal, in turn, controls the activity of target proteins with embedded cysteine residues by affecting their thiol–disulfide balance. The resulting changes in activity may impact the cellular processes affected by these proteins. Figure 8: Model for redox control of protein function in the cytosol. The cytosolic glutathione couple is positioned in vivo to sensitively amplify redox events affecting its oxidation state, via its redox potential E . This signal, in turn, controls the activity of target proteins with embedded cysteine residues by affecting their thiol–disulfide balance. The resulting changes in activity may impact the cellular processes affected by these proteins. Full size image The glutathione couple can be thought of as a broker that mediates the indirect effects of oxidants and reductants on the thiol–disulfide balance of many proteins. As the activity of proteins can be affected by this balance, the high sensitivity of E GSH to changes in glutathione oxidation may enable cells to respond to very small changes in the concentration of these reactive chemical species, well before their concentration is high enough to be toxic. This form of intracellular signalling may enable cells to mount an adaptive response to counteract the toxicity of a subsequent and more massive exposure to one of these reactive species. Indeed, disulfide bond formation in direct regulators of Nrf2 and NFκB increases transcription by these factors, which plays an important role in the cellular response to oxidants [7] , [45] . What would happen if the glutathione couple acted as a redox buffer? We expect that thiol–disulfide modification of in principle responsive proteins would become insensitive to redox events that affect the fraction of oxidized glutathione, as those events would no longer entail significant changes in redox potential. For example, the same change in glutathione oxidation that results in a 10 mV increase in E GSH when the couple is in a highly sensitive region of the Nernst curve ( OxD GSH =0.0019, GSH tot =10 mM) would only cause a 0.165 mV increase if the couple were optimally positioned as a buffer. As can be seen in Fig. 7 , under buffering conditions, such an event would no longer lead to a change in the thiol–disulfide balance of the protein network targeted by glutathione. As the glutathione couple is so abundant [1] , the concentration of GSSG in the cytosol remains significant compared with the typical concentrations of cytosolic proteins, even though most glutathione is in the reduced form. We estimate that GSSG concentration is about 9 μM in the average pm3 muscle of C. elegans ( OxD GSH =0.0019, assuming GSH tot =10 mM). This concentration is comparable to the 1 μM median concentration of cytosolic proteins in yeast [46] , [47] and is only slightly lower than the concentration of abundant cytosolic proteins (for example, the concentrations of ten glycolytic enzymes in mammalian muscle ranges between 29 and 131 μM [48] ). A 9 μM GSSG concentration is also much higher than the 0.001–0.7 μM physiological concentration range of cytosolic hydrogen peroxide in aerobic organisms [49] . Therefore, the kinetics of thiol–disulfide exchange between the glutathione couple and its target protein couples are not likely to be limited by the concentrations of GSSG and GSH. This means that the glutathione couple is well positioned to mediate efficiently the transfer of electrons to and from its target proteins. The differences in glutathione redox potential that we observe in the C. elegans pharynx reflect the population’s diversity rather than the individual’s variation over time, as individuals have essentially stable glutathione redox potentials over the course of almost an hour ( Supplementary Fig. 2 ). It is notable that individuals can exhibit distinct and stable glutathione redox potentials, as those differences must arise as a result of miniscule differences in glutathione oxidation. For example, the entire 12 mV range of pharyngeal E GSH values would be due to OxD GSH values between 0.0012 and 0.0028, assuming GSH tot =10 mM for all animals. This means that C. elegans is able to control glutathione oxidation with great precision. Thus, the thiol–disulfide balance of the network of protein targets of the glutathione couple is capable of both stability (as a result of the control of glutathione oxidation) and sensitivity (as a result of the high-sensitivity of glutathione redox potential to changes in glutathione oxidation). The vast majority of cytosolic glutathione (>99%) is found in the reduced state in a wide range of cell types and organisms [1] . For example, cytosolic OxD GSH is 0.00004 in yeast [43] , 0.0007 in cultured human HeLa cells [21] , [50] , 0.0066 in rat liver [1] and 0.009 in Escherichia coli [51] . When placed in the context of the Nernst curve, these OxD GSH values indicate that the glutathione couple is positioned in the highly sensitive, non-buffering region of the curve in all of these organisms ( Fig. 5 ). Thus, this property is not unique to C. elegans . In the C. elegans pharynx, variation in OxD GSH values between individuals leads to differences in the magnitude of their response to t -BuOOH treatment. Similarly, variation in OxD GSH values across species suggests large differences in redox sensitivity to changes in glutathione oxidation. For example, we predict yeast to be 159-fold more sensitive than rat liver cells to a small change in OxD GSH . It would be interesting to explore what adaptive constrains caused species to position their glutathione couple to provide different redox sensitivities. Although the glutathione couple facilitates a sensitive regulation of the thiol–disulfide balance of target proteins in the cytosol, it may well play a buffering role in other subcellular compartments. Redox potential is optimally buffered by the glutathione couple when OxD GSH equals 0.414 ( Fig. 5b ). This optimal value is in excellent agreement with measured OxD GSH values of 0.4 in the endoplasmic reticulum [41] , [50] . We conclude that unlike in the cytosol, the glutathione couple is positioned to buffer the thiol–disulfide balance of target proteins in the endoplasmic reticulum. The glutathione couple’s capacity to sensitively affect the thiol–disulfide balance of its target protein network may be advantageous by enabling organisms to respond to small perturbations to the cytosolic redox environment. However, this sensitivity could also amplify the effects of any breakdown in cellular redox homeostasis, setting the stage for the association between cytosolic redox changes and the aetiology and progression of many human diseases, particularly those for which ageing is a strong risk factor [9] , [10] , [11] . Strains and culture C. elegans were cultured under standard conditions at 20 °C. Wild-type C. elegans was Bristol N2. Construction of transgenes We built roGFP1_R12 from the vector pPD96_32 (Fire vector kit, Addgene), which contains a green fluorescent protein (GFP) construct optimized for expression efficiency in C. elegans . We replaced seven residues in this construct (C48S, C65S, S147C, N149K, S202K, Q204C and F223R) by site-directed mutagenesis (QuickChange, Stratagene) to generate roGFP1_R12 (ref. 23 ). We used a combination of classical cloning and fusion PCR to remove the mitochondrial-targeting sequence in the original plasmid and to fuse the roGFP1_R12 coding sequence to specific promoters. The fusion PCR for the coding region was done with 12 cycles of amplification to minimize the chances of introducing sequence errors (Expand High Fidelity PCR System, Roche), and cloned into a TOPO BluntII vector. We confirmed the sequence for all the constructs injected by DNA sequencing, using the primers listed in Supplementary Table 4 . roGFP1_R12 expression in pharyngeal muscle. We amplified the myo-2 promoter from pPD80.08 (Fire vector kit, Addgene) with primers WF45 and WF46, and cloned the PCR product into a TOPO BluntII vector. roGFP1_R12 was inserted into this vector backbone by restriction with Age I and Bswi WI, generating Pmyo-2::roGFP1_R12. roGFP1_R12 expression in intestine . We amplified the sur-5 promoter from pPD158.87 (Fire vector kit, Addgene) with primers WF45 and WF49, and cloned the PCR product into a TOPO BluntII vector. We fused this promoter to a restriction fragment containing roGFP1_R12 by secondary PCR using primers WF38 and WF129, generating Psur-5::roGFP1_R12 , which was cloned into a TOPO BluntII vector. Although we expected the sur-5 promoter to drive roGFP1_R12 expression in several tissues, we observed high expression of roGFP1_R12 only in the intestine at the × 100 magnification we used for imaging animals throughout this study. roGFP1_R12 expression in touch neurons . We amplified the mec-4 promoter from C. elegans genomic DNA with primers WF96 and WF99, and cloned the PCR product into a TOPO BluntII vector. roGFP1_R12 was inserted into this vector backbone by restriction with Age I and Pst I, generating Pmec-4::roGFP1_R12. Generation of transgenic animals and construction of strains The plasmids containing Pmyo-2::roGFP1_R12 and Pmec-4::roGFP1_R12 were microinjected using rol-6(su1006) as coinjection marker. The plasmid containing Psur-5::roGFP1_R12 was microinjected without a coinjection marker. Pmyo-2::roGFP1_R12 , Pmec-4::roGFP1_R12 and Psur-5::roGFP1_R12 were microinjected into wild type at concentrations ranging from 15 to 50 ng μl −1 , to generate ydEx20 and ydEx40 , ydEx37 and ydEx42 , and ydEx25 , ydEx22 and ydEx24 , respectively. ydEx20 was integrated into the genome by irradiation with ultraviolet light (254 nm), generating ydIs1 . After integration, the strain was outcrossed six times to wild type. Double and triple mutants were generated by standard genetic methods. Unless noted, measurements in pharynx, PLM neurons and intestine were performed in ydIs1 , ydEx37 and ydEx25 animals, respectively. gcs-1(ok436)/unc-4(e120) oxIs322[Cb-unc-119(+) , Pmyo-2::mCherry::H2B and Pmyo-3::mCherry::H2B] ; ydEx20 was derived by crossing gcs-1(ok436)/mIn1[mIs14 dpy-10(e128)] males with unc-4(e120) oxIs322; ydEx20 hermaphrodites. The 25 °C Daf-c phenotype was used to identify daf-2(e1370) and daf-2(m579) mutants. daf-16(mu86) and daf-16(+) were distinguished by PCR [33] . Transgenes were identified based on the presence of green fluorescence in the pharynx ( ydIs1 , ydEx20 and ydEx40 ), mechanosensory neurons ( ydEx37 and ydEx42 ) and intestine ( ydEx25, ydEx22 and ydEx24 ). oxIs322 was identified based on the presence of red fluorescence in the pharynx. Live microscopy We performed live fluorescence measurements in Petri dishes (50 × 9 mm, Falcon). We modified the standard NGM (Nematode Growth Media) to optimize imaging conditions. The modified media (which we refer as ‘NIM’, for Nematode Imaging Media) does not contain peptone and contains agarose instead of agar (to minimize the fluorescence of the media on illumination with 410 and 470 nm light); it also does not contain CaCl 2 (to prevent the formation of a precipitate that reduces light transmittance), nor cholesterol and MgSO 4 (normally included to support long-term nematode culture, but dispensable in the short time scales of imaging). The use of NIM resulted in 3.5- and 2.6-fold background reductions in the 410 and 470 nm channels, respectively. This optimized media produced background levels equal to only 1.6 and 1.4 times the camera noise in those channels. To prepare 100 ml of NIM, 2 g agarose and 0.3 g NaCl were dissolved in 96.5 ml of water and melted in a microwave. When the solution cooled down to 50 °C, we added 2.5 ml 1 M K 2 HPO 4 /KH 2 PO 4 pH 6.0 and 1 ml 0.5 M levamisole. We poured 7 ml of NIM per Petri dish, air dried the plates at room temperature for 1 h, stored them at 4 °C and used them within 2 weeks. Animals were staged by transferring 30 to 50 late L4 hermaphrodite larvae to NGM plates ( Figs 1 , 2 and 4a–c , and Supplementary Fig. 1 ); or NGM plates with 4.5 μg ml −1 5-fluoro-2′-deoxyuridine (Sigma, Figs 3 , 4d–e and 6 ), with each plate being considered as a technical replicate. For all experiments, at least two replicates per condition were considered during the same day of imaging, and measurements were performed in two different days at least, providing a minimum of four technical replicates. Imaging was conducted between 44 and 52 h after transfer (day 2 of adulthood), except for Fig. 1 and Supplementary Fig. 1 (day 1 of adulthood) and Supplementary Fig. 3 (L2 larval stage). Before imaging, worms were transferred to NIM plates at room temperature (21–23 °C) for 90 min. The imaging order between conditions was randomized. Imaging hardware and illumination Imaging was conducted on a motorized Axioskop 2 FS plus microscope (Zeiss) using a × 10 Plan-Apochromat 0.45 numerical aperture, 2-mm working distance objective lens (1063-139, Zeiss). Imaging plates were controlled by a motorized stage (ProScan II, Prior) with a stage-mounted customized Petri dish holder. Images were acquired with Metamorph 7.5.3.0 software. All microscopy was performed at 22 °C. Excitation at 410 and 470 nm was performed sequentially with a high-speed filter changer (Lambda DG-4, Shutter Instrument Company) controlling the excitation filters D410/30x and D470/20x. The filtered light was reflected by a 500dcxr dichroic mirror to illuminate the specimen. The emitted fluorescence passed through the filter HQ535/50m and was detected with a Cool SNAP HQ [2] 14-bit camera (Photometrics). All filters were manufactured by Chroma. Optimization of microscopy for different tissues We optimized exposure times to use at least two thirds of the dynamic range of the camera. This step ensures that image segmentation is performed consistently across all experimental conditions and for all imaged tissues, making the automatic image segmentation a blinded process for the researcher. We chose the camera binning based on the spatial resolution required for tissues of different morphology and size. To image the feeding muscles of the pharynx, we focused on the plane of the pharyngeal lumen under transmitted light. Fluorescence images were acquired with 4 × 4 binning using an average exposure time of 40 ms ( Figs 1 , 2 , 4 and 6 ). Higher spatial resolution images were acquired with 2 × 2 binning, with average exposure times of 165 ms and 300 ms, respectively for Fig. 3 and Supplementary Fig. 3 . In control experiments, we imaged 20 animals sequentially with 2 × 2 and 4 × 4 binning, and found that the resulting estimates of the ratio of fluorescence ( R 410/470 ) are highly correlated ( r =0.961, P <0.0001). To image the intestine, we concentrated on the posterior region of the tissue, which exhibits higher sensor expression. Fluorescence images were acquired with 4 × 4 binning, using average exposure times of 105 ms. To image mechanosensory neurons, we selected the PLM neurons because they are located at the tail of the worm were the specimen is thin and flat and, therefore, short focal depth is required for imaging. Only one of the two PLM neurons was quantified for each worm. Fluorescence images were acquired with 2 × 2 binning using average exposure times of 450 ms. Image processing and segmentation Image processing was conducted in ImageJ (NIH) and Matlab (Mathworks). We performed background subtraction by removing the mode intensity value of the entire image from each pixel. This procedure removes the background due to the agar and the camera noise, as the vast majority of pixels in our images were part of the background. To segment the images, we defined regions of interest (ROI) by applying a threshold in the 410 nm excitation images. We used the same intensity value for the segmentation across all tissues and conditions. In the case of the PLM neurons, the ROIs correspond to single cells; in the case of the intestine, the ROIs correspond to the most posterior portion of the tissue (~85 μm in length); in the case of feeding muscles, the ROIs correspond to the entire pharynx. We used the ROIs to quantify both the 410 and 470-nm excitation images ( I 410 and I 470 images, respectively). We obtained nearly identical R 410/470 values by segmenting based on I 410 or I 470 images ( r =0.999, P <0.0001, for the individuals in Fig. 3 ). Ratiometric measurements We calculated R 410/470 by computing the ratio of the total fluorescence between the segmented I 410 and I 470 regions. To study how R 410/470 and its transforms vary along the A–P axis of the pharynx, we generated R 410/470 profiles along the midline of this tissue using automated scripts in ImageJ. First, the segmented I 410 and I 470 regions were rotated, centred and reflected to orient them along their A–P axis. We then constructed a polyline in the I 410 image along the midline of the pharynx using features of five morphological pharyngeal landmarks. This polyline was visually inspected and, when necessary, adjusted manually to ensure the quality of the alignment to the midline of each pharynx. We refer to this polyline as the ‘medial axis of the pharynx’, and measurements conducted along the medial axis as ‘anterior–posterior pharyngeal profiles’. We measured the intensity along the medial axis in I 410 and I 470 images, using a line width of 5.16 μm (2 pixels) for 4 × 4 binning images and using a line width of 7.74 μm (6 pixels) for 2 × 2 binning images. The resulting intensity vectors were then length normalized using bilinear interpolation. We determined the E profile along the A–P axis of the pharynx from the computed element-wise intensity ratios ( I 410 / I 470 ) between these two vectors. We note that the average value of E for the medial axis (computed from the ratio of 410 to 470 total fluorescence along the medial axis) approximates very closely that of the whole pharynx ( r =0.9988, P <0.0001 for the 394 animals in Fig. 3 ). To calculate the value of E for individual muscle segments, we identified muscle boundaries based on the position of the morphological landmarks of the pharynx in the length-normalized intensity vectors. We computed E from the ratio of the 410 and 470 nm total intensities within each region. Image visualization Pixel-by-pixel E images, computed from the raw unsegmented I 410 and I 470 images, provide a valuable visualization tool that complements the formal image analysis and quantification described above. We computed E from pixel-by-pixel R 410/470 values and generated red, green, and blue (RGB) images by mapping E values to a colormap. We wanted these images to provide information about the magnitude of the intensity signals used, de-emphasizing pixels where the signal was low. To this end, we adjusted the brightness of pixels whose intensity values in the I 410 or I 470 images were below the value of the intensity cutoff used for segmentation (equal to 2,000 in all images shown). Images were transformed to the hue-saturation-brightness colour space and pixels with intensity values above the cutoff were assigned a brightness value of 1, while those with intensities below the cutoff were assigned a brightness value equal to their intensity divided by the cutoff value. The resulting hue-saturation-brightness image was transformed to RGB for visualization. We used the cool–warm and similar diverging colormaps [52] to colour-code images and pharyngeal E profiles, as these colormaps are perceptually linear and behave well for observers with colour-deficient vision. Determination of OxD roGFP and E roGFP from R 410/470 To calculate the fraction of roGFP1_R12 molecules with a disulfide bond ( OxD roGFP ) from ratiometric fluorescence measurements [17] , we determined empirically the value of the three parameters relating OxD roGFP to R 410/470 , as described in the legend of Fig. 1 . We note that the parameter α determines the curvature of the relationship from R 410/470 to OxD roGFP (if α were equal to 1, then the relationship in Fig. 1e would be linear).We treated worms with various concentrations of oxidants and reductants, and found that the sequential treatment with the oxidant diamide (50 mM, Sigma) followed by treatment with the reducing agent DTT (100 mM, Sigma), resulted in maximal oxidation and reduction of the sensor, respectively, in the pm3 muscles of the pharynx. The in vivo dynamic range of the sensor matched the reported in vitro dynamic range [23] . These experiments also showed that 50 mM diamide treatment and 100 mM DTT treatment affect the expression of the roGFP1_R12 sensor and GFP S65C by at most 10%, in the timescale of the Fig. 1 experiment. All chemical incubations were performed in NIM plates. No photobleaching was observed during incubations. We calculated the potential of the redox couple defined by oxidized and reduced forms of roGFP1_R12 using the Nernst equation E = E roGFP °′ —[ RT /(2 F )] ln [(1- OxD roGFP )/ OxD roGFP ], with the standard roGFP1_R12 half-cell reduction potential ( E roGFP °′ ) of −265 mV [23] , a temperature of 295.15 °K (22 °C) and assuming a cytosolic pH of 7. The final relation from R 410/470 to E roGFP is given by the expression E roGFP = E roGFP °′ −[ RT /(2 F )] ln {[ α ( R ox − R 410/470 ) ]/( R 410/470 − R red )}. It is noteworthy that the parameter α shifts E roGFP by a constant value equal to −[ RT /(2 F )] ln α . As a result, E roGFP differences are not affected by this parameter. We also note that although the value of E roGFP is influenced by pH (by shifting the midpoint potential of the couple), under physiological conditions these effects are not relevant to understand the equilibration of potentials between roGFP1_R12 and glutathione couples [1] , [17] . This is because both couples involve the exchange of two protons and two electrons and, under physiological conditions, pH is well below the p K a of the reactant thiols (p K a =8.92 for GSH and ~9.0 for roGFP1_R12 C147 and C204); as a result, the midpoint potentials of these redox couples are affected by pH in the same direction and by essentially the same amount [17] , [23] , [53] . We also note that the fluorescence ratio emitted by roGFP1 is unaffected by changes in pH in the physiological range (6.0–8.5) [19] , which encompass the reported 6.9–7.5 range in cytosolic pH of C. elegans intestine and 7.5 cytosolic pH of C. elegans body muscle [54] , [55] . Ratiometric measurements in gcs-1 mutants The gcs-1(ok436)/unc-4(e120) oxIs322 ; ydEx20 strain was used as a parental strain in experiments with the gcs-1 mutant. gcs-1(ok436) homozygous progeny from that strain were identified by the lack of mCherry pharyngeal expression. These gcs-1(maternal+zygotic−) animals arrested during larval development. Their gcs-1(maternal+zygotic+) siblings expressed mCherry in the pharynx and did not arrest larval development. Ratiometric measurements were performed in pm3 muscles at the L2 larval stage. tert -butyl hydroperoxide assays We treated animals with 5 mM t -BuOOH, in freshly made imaging plates (used within 4 h of preparation). R 410/470 time series in untreated individual worms were acquired for 10 min before t -BuOOH treatment. Individual worms were then transferred to plates with 5 mM t -BuOOH and imaged for additional 60 min, with a gap of 3–6 min between treatments. Images were acquired every 30 s. Statistical analysis All statistical analyses were performed in JMP (SAS) and Matlab (Mathworks). We tested for differences in the average E among groups using analysis of variance. We used the Tukey HSD post-hoc test to determine which pairs of groups in the sample differ, in cases where more than two groups were compared. We used least-squares regression to quantify genetic interactions between wild-type and mutant alleles of daf-2 and daf-16 using the following linear model: E =Intercept+ daf-2 + daf-16 + daf-2 * daf-16+ε . The second to last term in this model quantifies the existence, magnitude and type (synergistic or antagonistic) of genetic interaction between daf-2 and daf-16 mutant alleles. Functional data analysis We used the functional data analysis statistical package in Matlab [56] to model and analyse positional series of E -values in pharyngeal A–P profiles and time series of E -values in the response to t -BuOOH. The basic idea of this approach is to express discrete spatial or temporal series of observations in the form of a function. These functions are then treated as single observations, which are analysed statistically applying concepts of multivariate analysis [34] . A more detailed description of our application of this technique is given in the Supplementary Methods . How to cite this article: Romero-Aristizabal, C. et al. Regulated spatial organization and sensitivity of cytosolic protein oxidation in Caenorhabditis elegans . Nat. Commun. 5:5020 doi: 10.1038/ncomms6020 (2014).